Interconvertible vanadium-seamed hexameric pyrogallol[4]arene nanocapsules Research into stimuli-responsive controlled self-assembly and reversible transformation of molecular architectures has received much attention recently, because it is important to understand and reproduce this natural self-assembly behavior. Here, we report two coordination nanocapsules with variable cavities: a contracted octahedral V 24 capsule and an expanded ball-shaped V 24 capsule, both of which are constructed from the same number of subcomponents. The assemblies of these two V 24 capsules are solvent-controlled, and capable of reversible conversion between contracted and expanded forms via control of the geometries of the metal centers by association and dissociation with axial water molecules. Following such structural interconversions, the magnetic properties are significantly changed. This work not only provides a strategy for the design and preparation of coordination nanocapsules with adaptable cavities, but also a unique example with which to understand the transformation process and their structure-property relationships. The design and synthesis of discrete metal-organic nanocapsules (MONCs) with specific geometries and cavities have been investigated extensively due to not only their interesting structures [1] , [2] , [3] , but also their promising applications in supramolecular chemistry [4] , [5] , [6] and material science [7] , [8] , [9] . To date, a large number of MONCs have been synthesized from metal ions or metal clusters with different coordination environments and organic linkers with various shapes [10] , [11] , [12] . Of particular recent interest is control of the self-assembly of the MONCs by external stimuli [13] , [14] including light [15] , [16] , electricity [17] , pH [18] , guests [19] , and solvents [20] . Studies of this self-assembly may help us to understand and further mimic stimuli-responsive structural reorganization processes in biological systems. However, the structural transformations of the reported stimuli-responsive MONCs are usually accompanied by major changes in the species and number of subcomponents including metal centers and ligands. In contrast, exploration of stimuli-responsive MONCs with equal subcomponents [21] , [22] , or MONC quasi-isomers [23] , [24] with the same metal centers, but some different coordinated components [15] , [16] , which act similarly to natural macromolecules is still in its infancy. Recognition of the reversible structural interconversion between such isomers or quasi-isomers will not only provide new approaches to broaden the preparation of MONCs with different shapes, but also an understanding of their structure–property relationships, such as host–guest recognition, drug delivery and release, and supramolecular catalysis [16] , [25] , [26] . C-alkylpyrogallol[4]arenes (abbreviated as PgC n , where n is the length of the associated alkyl tail), which are vase-shaped macrocyclic host molecules composed of 1,2,3-trihydroxybenzene units, have been determined over the past decade to be versatile building blocks for the construction of supramolecular complexes [27] . For example, PgC n can assemble itself to form isolated MONCs [28] , [29] , hydrogen-bonded capsules [30] , [31] , hydrogen-bonded/metal-organic nanotubes [32] , [33] , and supramolecular organic frameworks [34] . Since the initial discovery by Atwood et al. in 2005 [35] of PgC n -based MONCs constructed from six PgC n units and 24 Cu 2+ ions, a number of studies have demonstrated that PgC n can self-assemble into octahedral hexameric M 24 (M=Mg, Co, Ni, Cu, and Zn) [36] , [37] , [38] , [39] , [40] , spherical dimeric M 8 (M=Co, Ni, Cu, and Zn) [41] , [42] , [43] , “rugby ball” shaped hexameric Ga 12 [44] or mixed nanocapsules [45] , [46] , [47] . Interestingly, spherical Cu 8 and Zn 8 dimers can be linked by 4,4′-bipyridine ligands into a one-dimensional coordination polymer [48] and an MOF-like structure [49] , respectively. However, PgC n -based MONCs are limited to the aforementioned metal ions, and still have the possibility of synthesizing new PgC n -based MONCs and exerting control over their self-assembly behavior. Vanadium is of particular interest in this context owing to its various coordination behaviors, valence states, and promising applications in areas such as magnetism [50] , [51] , [52] , optics [53] , and catalysis [54] . Currently, the number of known vanadium capsules is limited [55] , [56] , [57] , [58] and here we report an interesting example of solvent-responsive assembly of coordination nanocapsule quasi-isomers with distinct geometries. This includes a contracted octahedral capsule (V 24 -oct) with the inner cavity of 1000 Å 3 , and an expanded ball-shaped capsule (V 24 -ball) with inner cavity of 1400 Å 3 , from the same number of subcomponents including 24 vanadium centers and 6 pyrogallol[4]arene units (Fig. 1 ). These two V 24 capsules represent an example of a metal displaying versatility and forming different PgC n -based hexamer capsules. Fig. 1 Controlled self-assembly and interconversions of V 24 capsules. Chemical structure of hexameric pyrogallol[4]arene V 24 octahedron and V 24 ball from 6 PgC 3 ligands and 24 vanadium ions. Vanadium is green, oxygen red and carbon blue Full size image Synthesis and characterization of V 24 octahedron and ball C -Propylpyrogallol[4]arene (PgC 3 , Fig. 1 ) was synthesized as reported by Gerkensmeier et al. [59] by a condensation reaction of pyrogallol and butanal catalyzed by concentrated hydrochloric acid. The reaction of PgC 3 with VOSO 4 ·5H 2 O in CH 3 CN/H 2 O solution (10:1, v/v) at 80 °C for three days yields green rhombic crystals of V 24 -oct-α with the formula [V 24 O 24 (H 2 O) 24 (C 40 H 40 O 12 ) 6 ]∙(solvent) x . Single-crystal X-ray diffraction analysis shows that the V 24 -oct-α crystallizes in the trigonal system with space group R -3 and consists of 6 PgC 3 units and 24 V ions arranged in 8 trinuclear V 3 clusters capping the face of the octahedron (Fig. 2a ). The overall geometry of this capsule is similar to the previously reported octahedral hexameric M 24 (M=Mg, Cu, Co, Ni, and Zn) capsules [36] , [37] , [38] , [39] , [40] . Inspection of the crystal structure of V 24 -oct-α reveals that each V 3 cluster is held together by three pyrogallol (Pg) units from different bowl-shape PgC 3 ligands (Fig. 2b ). The angle between the two opposite upper-rim oxygen atoms and the lower-rim centroid at the base of the PgC 3 ligand is about 108.9° and the separation between two opposite faces of the octahedron, measured from the opposite centroids of the V 3 clusters is approximately 14.3 Å (Supplementary Figures 4 and 5 ). These three V centers adopt octahedral geometries, and each one is coordinated with four phenoxyl oxygen atoms from two different PgC 3 ligands, one interior water molecule, and one exterior oxygen atom (Fig. 2c ). Further analysis shows that three V centers, situated at the vertices of an approximately equilateral triangle, in which V···V distances are in the range of 3.752–3.763 Å, are linked by three phenoxyl oxygen atoms to form a planar V 3 O 3 array. In this array, the V···O distances range from 1.987–2.001 Å, the O−V−O angles range from 98.18–99.09°, and the V−O−V angles range from 140.08–141.17°. The capsule contains an internal cavity with a volume of ~ 1000 Å 3 , calculated using VOIDOO with a probe radius of 1.2 Å. 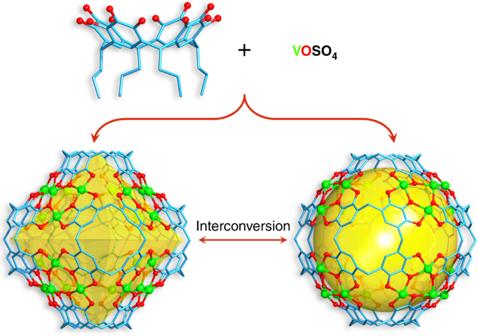Fig. 1 Controlled self-assembly and interconversions of V24capsules. Chemical structure of hexameric pyrogallol[4]arene V24octahedron and V24ball from 6 PgC3ligands and 24 vanadium ions. Vanadium is green, oxygen red and carbon blue 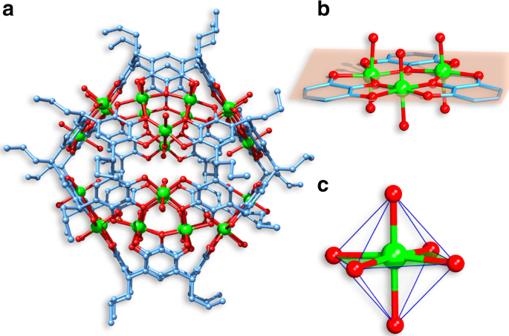Fig. 2 Structural representations of V24-oct-α from X-ray diffraction data.aMolecular structure of V24-oct-α.bMetal-ligand arrangement andccoordination geometries of V ions within the capsule Bond valence sum (BVS) calculations and EPR analysis reveal that the vanadium centers in V 24 -oct-α are at +4 oxidation states (Supplementary Table 2 and Supplementary Figure 1 ). In addition, the IR spectrum of V 24 -oct-α shows the characteristic V═O band in the frequency range 950–990 cm −1 (Supplementary Figure 2 ). It is interesting that the introduction of N , N -dimethylformamide (DMF) to the reaction of V 24 -oct-α produces its polymorph V 24 -oct-β which crystallizes in the triclinic space group P- 1. Fig. 2 Structural representations of V 24 -oct-α from X-ray diffraction data. a Molecular structure of V 24 -oct-α. b Metal-ligand arrangement and c coordination geometries of V ions within the capsule Full size image Interestingly, changing the CH 3 CN/H 2 O solvent in the preparation of V 24 -oct-α to NMF/CH 3 OH (1:1, v/v; NMF= N -methylformamide) affords green tetragonal prism crystals of V 24 -ball-β: [V 24 O 24 (C 40 H 40 O 12 ) 6 ]∙(solvent) x , which crystallizes in the tetragonal space group P 4/ mnc and contains the same number of components as V 24 -oct-α (Fig. 3a ). This capsule can be regarded as an expanded structure of the V 24 -oct-α for two main reasons. The angle between the two opposite upper-rim oxygen atoms and the lower-rim centroid at the base of the PgC 3 ligand has expanded to 123.1° and the separation between two opposite centroids of V 3 clusters in this ball increases to 16.7 Å, compared to V 24 -oct-α (Supplementary Figures 4 and 5 ). As a result of these expansions, the inner cavity volume of the V 24 -ball-β increases to ~ 1400 Å 3 , which is ~ 400 Å 3 larger than the cavity in V 24 -oct-α. Upon close examination, their structural transformations can be seen to be due to the coordination geometry differences in V centers. In this case, all the V ions are five-coordinated in square-pyramidal coordination geometries and coordinated by four phenoxyl oxygen atoms from two different PgC 3 ligands and one exterior oxygen atom (Fig. 3c ). The changes of coordination geometry in the V ions have a large influence on the bond angles and the shape of the V 3 O 3 array from the aforementioned V 24 -oct-α. Specifically, the V 3 O 3 array in V 24 -ball-β is concavoconvex with V···O distances ranging from 1.953–2.037 Å, O−V−O angles ranging from 88.52–89.43°and V−O−V angles ranging from 134.38–137.12° (Fig. 3b ). Except for the V···O distances, it is clear that the O−V−O and V−O−V angles in this capsule are much smaller than those in V 24 -oct-α quasi-isomer. 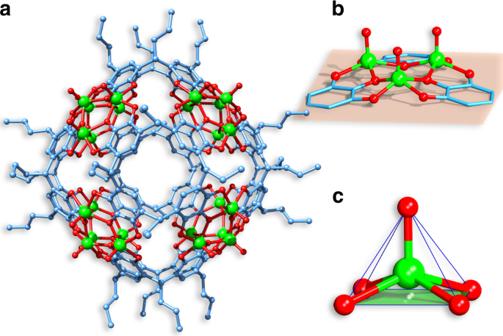Fig. 3 Structural representations of V24-ball-β from X-ray diffraction data.aMolecular structure of V24-ball-β.bMetal-ligand arrangement andccoordination geometries of V ions within the capsule BVS calculations and EPR analysis together with IR spectra reveal that the vanadium centers in V 24 -ball-β are at +4 oxidation states with a VO 2+ form (Supplementary Table 3 and Supplementary Figures 1 and 3 ), which are the same to those in V 24 -oct-α. Whereas the structural differences in previously reported MONC isomers and quasi-isomers arise from the plasticity of the ligands [15] , [16] , [21] , [22] , these two different types of V 24 capsules represent an example of MONC quasi-isomers whose structural differences stem from the coordination diversity of metal centers. By replacing the NMF with DMF in the same reaction, its polymorph V 24 -ball-α was obtained and was found to crystallize in a cubic system with the space group Ia- 3. Fig. 3 Structural representations of V 24 -ball-β from X-ray diffraction data. a Molecular structure of V 24 -ball-β. b Metal-ligand arrangement and c coordination geometries of V ions within the capsule Full size image Interconversions between V 24 capsules It has been observed that the five-coordinate square pyramidal and six-coordinated octahedral oxidovanadium complexes can interconvert by associating and disassociating an axial molecule [60] , [61] , [62] . With this in mind, we searched for conditions which promote the interconversion between the contracted V 24 octahedron and the expanded V 24 ball. Interestingly, we found that the axial water molecules of vanadium centers in V 24 octahedron are removed in DMF/CH 3 OH (1:1, v/v) solution at 80 °C, the DMF working as a dehydrating agent; [63] while those vanadium centers in V 24 ball-shaped capsule can capture the water molecules in DMF/CH 3 CN/H 2 O/NEt 3 (20:80:10:1, v/v/v/v) solution at 80 °C (Fig. 4 ). The dissociation and association of axial water molecules in vanadium centers lead to their coordination geometries changing from square pyramidal and octahedral forms (Fig. 2c and Fig. 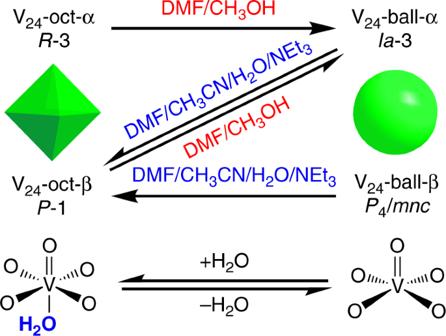Fig. 4 The transformation mechanism of V24capsules. The transformation mechanism of V24octahedron and ball can be achieved by controlling the geometries of vanadium ions by association and dissociation with axial water molecules in different solvent conditions 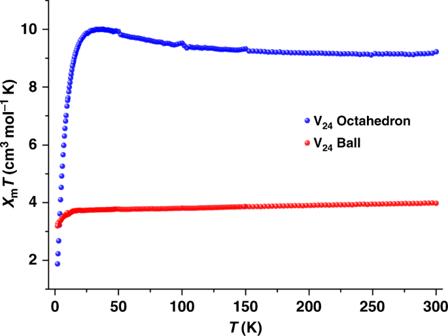Fig. 5 Magnetic data for V24capsules. Plots ofχmT vs. T for V24-oct-α and V24-ball-β in a 1 kOe field 3c ), respectively. When the vanadium centers adopt octahedral geometry, they and the equatorial coordinated oxygen atoms from the Pg units are almost coplanar (Supplementary Figure 6a ). In contrast, when adopting square-pyramidal geometries, the vanadium ions and those oxygen atoms form a curved surface (Supplementary Figure 6b ). Such transformations between the plane and curved surfaces result in the changes of inner cavities from contracted octahedra to an expanded ball in V 24 capsules. As shown in Fig. 4 , V 24 -oct-α and V 24 -ball-β can be easily converted into V 24 -ball-α and V 24 -oct-β, respectively, but the reverse is not observed. However, V 24 -oct-β and V 24 -ball-α can interconvert by regulating the solvents, which leads to form the V 24 capsule partners showing different shapes. To sum up, the interconversions between the contracted and expanded V 24 capsules have been successfully achieved by a process involving dissolution-reaction-recrystallization, which has been found to be an excellent method to explore the structural transformation of isolated coordination compounds as well as MONCs [64] , [65] , [66] . However, attempts to achieve the transformations through single-crystal-to-single-crystal phase transition under the stimulation of temperature and pressure were hindered by poor crystal quality, because packing of these V 24 capsules is via weak supramolecular interactions, and the crystals of V 24 capsules easily lose crystallinity after partial loss of the solvent. Fig. 4 The transformation mechanism of V 24 capsules. The transformation mechanism of V 24 octahedron and ball can be achieved by controlling the geometries of vanadium ions by association and dissociation with axial water molecules in different solvent conditions Full size image Magnetic properties of V 24 capsules Given the structural differences between these two V 24 capsules, we compared their magnetic properties in order to yield important prototypes for exploring structure–property relationships. Here for clarity, we have provided only two phases (V 24 -oct-α and V 24 -ball-β) as examples, because the χ m T vs. T data for V 24 -oct and V 24 -ball with two different phases show similar trends (Fig. 5 and Supplementary Figure 7 ). The magnetic property analyses of these two V 24 capsules were performed on fresh samples from 2–300 K under a magnetic field of 1 kOe. For V 24 -oct-α, the room temperature χ m T value of 9.23 cm 3 ·K·mol −1 is close to the expected value of 9 cm 3 ·K·mol −1 for 24 spin-only V 4+ centers [50] , [51] , [52] . The value increases continuously with decreasing temperature, reaching a maximum of 10.01 cm 3 ·K·mol −1 at 35 K and subsequently decreases sharply to 1.88 cm 3 ·K·mol −1 at 2.0 K. The increase of the value of χ m T upon reduction of the temperature at higher temperatures indicates intramolecular ferromagnetic exchange between neighboring metal ions. The 35–300 K magnetic data of this capsule was fitted to the analytical experimental equation (Eq. 1 ) deduced for compounds with three spin centers in an equilateral triangle [67] , assuming the eight V 3 clusters are noninteracting: 
    χ_m = Nβ^2g^2/4kT1 + 5exp(3J/2kT)/1 + exp(3J/2kT)
 (1) Fig. 5 Magnetic data for V 24 capsules. Plots of χ m T vs . T for V 24 -oct-α and V 24 -ball-β in a 1 kOe field Full size image In Eq. 1 , N is Avogadro’s number, β is Bohr’s magneton and k is Boltzmann’s constant. The best exchange interaction parameters obtained from fitting the χ m data are J / k = 12.38 K and g = 1.93 (Supplementary Figure 8 ). The positive J value further suggests an intramolecular ferromagnetic interaction in V 24 -oct-α at higher temperatures. For the V 24 -ball-β, the room temperature value of χ m T of 3.97 cm 3 ·K·mol −1 is much lower than the expected value (9 cm 3 ·K·mol −1 ) for 24 spin-only V 4+ centers. This decreases gradually to 3.72 cm 3 ·K·mol −1 at ~ 20 K and then decreases rapidly reaching a value of 3.19 cm 3 ·K·mol −1 at 2 K. Analysis of the V 24 -oct-α using the same equation (Eq. 1 ) yields J/k = −653.8 K and g = 2.04 (Supplementary Figure 9 ). Both the curve and negative J indicate dominant antiferromagnetic exchange interactions within this capsule since χ m T at 300 K is much smaller than the expected values from 24 isolated V 4+ spin carriers [68] . Notwithstanding all V centers being at +4 oxidation states in both V 24 capsules, the variations between the five-coordinated square-pyramidal geometries in the V 24 -ball-β and the six-coordinated octahedral geometries in the V 24 -oct-α are indicative of a sensitive magnetic behavior of V 4+ centers in different ligand field environments. Neither an obvious hysteresis loop or peaks for the out-of-phase component are observed for both capsules (Supplementary Figures 10 - 13 ), and this reveals no single molecule magnetic behavior above 2 K for both capsules. We have developed a strategy for the efficient construction of MONC quasi-isomers by controlling the coordination environments of the metal centers. In the present case, the adoption of octahedral and square-pyramidal geometries of vanadium centers results in a contracted V 24 octahedron and an expanded V 24 ball, respectively. V 24 -oct-β is the key motif in the interconversion between the contracted and expanded V 24 capsules, which can be obtained by introducing DMF to the reaction of V 24 -oct-α and can also be prepared from V 24 -ball. The interconversions between V 24 -oct-β and V 24 -ball-α achieved by regulating solvents, leads to formation of the V 24 capsule partners with different shapes. This work thus represents an example of MONCs whose structural differences arise from the coordination diversity of metal centers. Materials and equipment All reagents and solvents used in synthetic studies were obtained from commercial sources and employed without further purification. IR spectra were recorded in the range 4000−400 cm −1 with a Magna 750 IR spectrometer using KBr pellets. Electron paramagnetic resonance (EPR) spectra were recorded on a Bruker ER-420 spectrometer with a 100 kHz magnetic field in the X band at room temperature. Magnetic susceptibilities were determined on a Quantum Design PPMS-9T and MPMS-XL systems in the range of 2–300 K. All experimental magnetic data were corrected for the diamagnetism of the sample holders and of the constituent atoms according to Pascal’s constants. IR, EPR spectra and magnetic data were measured on the V 24 -oct-α and V 24 -ball-β samples. Synthesis of PgC 3 ligand A solution of pyrogallol (20 g, 160 mmol) in ethanol (100 mL) and concentrated hydrochloric acid (10 ml) was mixed dropwise with butyraldehyde (11.4 g, 160 mmol) under N 2 gas. This mixture was heated to reflux for 24 h, cooled, filtered, washed with water, a little cold ethanol and dried under vacuum. PgC 3 was collected as a colorless powder. (13.6 g, 47%). 1 H NMR (400 MHz, acetone- d 6 ,): δ=0.95 (12H, t, CH 3 ), 1.31 (8H, m, CH 2 ), 2.26 (8H, q, CH 2 ), 4.35 (4H, t, CH), 7.14 (4H, s, ArH), 7.18 (4 H, s, OH), 8.09 (8H, brs, OH) ppm. Synthesis of V 24 octahedron Method 1: VOSO 4 ·5H 2 O (0.4 mmol) and PgC 3 (0.1 mmol) were added to CH 3 CN (5 mL), H 2 O (0.5 ml) and NEt 3 (50 μL). The mixture was sealed in an 8 mL glass vial, which was heated at 80 °C for three days, affording the green rhombic crystals of V 24 -oct-α with a low yield (8% based on the PgC 3 ligand). Enhancement of the synthetic yield can be achieved by the slow concentration of the filtrate at room temperature for one week, and in this way, the total yield of V 24 -oct-α was subsequently raised to 68%. Method 2: VOSO 4 ·5H 2 O (0.4 mmol) and PgC 3 (0.1 mmol) were added to DMF (1 mL), CH 3 CN (4 mL), H 2 O (0.5 ml) and NEt 3 (50 μL). The mixture was sealed in an 8 mL glass vial, which was heated at 80 °C for 24 h. After slow concentration of the filtrate at room temperature for one week, green block crystals of V 24 -oct-β were collected in ~ 72% yield according to the PgC 3 ligand. Synthesis of V 24 ball Method 1: VOSO 4 ·5H 2 O (0.4 mmol) and PgC 3 (0.1 mmol) were added to DMF (2 mL) and CH 3 OH (2 mL). The mixture was sealed in an 8 mL glass vial, which was heated at 80 °C for 24 h. After slow concentration of the filtrate at room temperature for five days, cubic crystals of V 24 -ball-α were collected in ~ 76% yield based on the PgC 3 ligand. Method 2: VOSO 4 ·5H 2 O (0.4 mmol) and PgC 3 (0.1 mmol) were added to NMF (2 mL) and CH 3 OH (2 mL). The mixture was sealed in an 8 mL glass vial, which was heated at 80 °C for 24 h. After slow concentration of the filtrate at room temperature for five days, green tetragonal prism crystals of V 24 -ball-β were collected in ~ 88% yield based on the PgC 3 ligand. Conversion from V 24 octahedron to V 24 ball In an 8 mL glass vial, synthesized crystals of V 24 -oct-α (10 mg) or V 24 -oct-β (10 mg) were dissolved in DMF (1 mL) and CH 3 OH (1 mL), and the mixture was heated at 80 °C for 48 h. The solution was allowed to stand at room temperature for ten days to obtain ~ 8.5 mg green cubic crystals of V 24 -ball-α, 81% yield. Conversion from V 24 ball to V 24 octahedron In an 8 mL glass vial, synthesized crystals of V 24 -ball-α (15 mg) or V 24 -ball-β (15 mg) were dissolved in DMF (0.5 mL), CH 3 CN (2 mL), H 2 O (0.25 ml) and NEt 3 (25 μL), and the mixture was heated at 80 °C for 48 h. The solution was allowed to stand at room temperature for one week to obtain ~ 12 mg green block crystals of V 24 -oct-β, 83% yield. Single crystal X-ray diffractions All X-ray single crystal data for V 24 capsules were measured on diffractometers equipped with copper micro-focus X-ray sources ( λ = 1.5406 Å) at 100.0(2) K. Diffraction data from V 24 -oct-α, V 24 -ball-β and V 24 -ball-α were measured on a SuperNova diffractometer, and that from V 24 -oct-β was collected on Bruker APEX-II CCD. The crystal structures were resolved by direct methods and all calculations were performed on the SHELXTL -2016 program package [69] . All non-hydrogen atoms were refined anisotropically with the exception of several highly disordered propyl carbon atoms and water molecules. Hydrogen atoms of the organic ligands were added in the riding model and refined with isotropic thermal parameters. Because of the diffuse electron density and the highly disordered/amorphous solvents, molecules of crystallization could not be fully located and were therefore not included for all structures (details are also provided in Supplementary Note 1 ). The crystal structures were treated by the “SQUEEZE” routine [70] , a part of the PLATON package of crystallographic software, dramatically improving the agreement indices. We attempted to finish the refinement, but the R 1 and wR 2 factors were still high and some A-alerts were found by the (IUCr) checkCIF routine, all of which could be ascribed to the weak crystal diffraction, which is typical in giant supramolecular assemblies. Details on crystal data collection and refinement for these capsules are summarized in Supplementary Table 1 .